A high-rate and long cycle life aqueous electrolyte battery for grid-scale energy storage New types of energy storage are needed in conjunction with the deployment of solar, wind and other volatile renewable energy sources and their integration with the electric grid. No existing energy storage technology can economically provide the power, cycle life and energy efficiency needed to respond to the costly short-term transients that arise from renewables and other aspects of grid operation. Here we demonstrate a new type of safe, fast, inexpensive, long-life aqueous electrolyte battery, which relies on the insertion of potassium ions into a copper hexacyanoferrate cathode and a novel activated carbon/polypyrrole hybrid anode. The cathode reacts rapidly with very little hysteresis. The hybrid anode uses an electrochemically active additive to tune its potential. This high-rate, high-efficiency cell has a 95% round-trip energy efficiency when cycled at a 5C rate, and a 79% energy efficiency at 50C. It also has zero-capacity loss after 1,000 deep-discharge cycles. The increasing deployment of renewable energy sources such as solar and wind power requires a commensurate increase in energy storage capacity to integrate them into the electrical power grid [1] , [2] . Combining these sources with the energy grid is especially challenging because of the large, rapid variability in their output. Intermittent spikes or drops in power must be smoothed for durations as short as a few seconds, whereas load balancing is needed to counter diurnal fluctuations [1] , [3] . Inexpensive energy storage that has rapid response, long cycle life, high power and high energy efficiency that can be distributed throughout the grid is needed to allow broad penetration of solar, wind and other variable energy sources. Conventional energy storage technologies struggle to meet the needs of the grid [2] . Virtually, all of the energy storage capacity currently on the grid is provided by pumped hydroelectric power, which requires an immense capital investment, is location-dependent and suffers from low energy efficiency [1] , [4] . Compressed air energy storage is also site-dependent and must be supported by a fossil fuel-burning plant. Mechanical flywheels offer high power and efficiency, but they are far too expensive. Several battery technologies have seen limited deployment on the grid [4] , [5] . Lead acid cells are the least expensive, but have limited depth of discharge, cycle life and efficiency. Sodium–sulphur, sodium–metal halide and redox-flow batteries operate only at low rates and have low energy efficiencies. Finally, the lithium ion and nickel/metal hydride batteries used in electric vehicles are currently far too costly for use on larger scales. A variety of novel aqueous alkali-ion battery chemistries have been explored in recent years. They are potentially advantageous owing to the safety, high ionic conductivity and low cost of aqueous electrolytes. Aqueous lithium-ion batteries using cathode materials adopted from commercialized organic electrolyte cells have been explored, but in general they have shown limited cycle life [6] , [7] , [8] . Aqueous sodium cells using a Na x MnO 2 cathode and a capacitive carbon anode have been demonstrated to offer long cycle life, but have limited rate capability [9] , [10] . These aqueous battery technologies have been limited primarily by the development of anode materials that have the correct potential and that are chemically stable at the desired electrolyte pH [11] . Recently, we developed a family of open-framework nanoparticle materials with the Prussian Blue crystal structure [12] , [13] , [14] , [15] . These materials have an open-framework crystal structure containing large interstitial sites that allows fast insertion and extraction of Na + and/or K + with very little crystallographic lattice strain. For example, copper hexacyanoferrate (CuHCF) reacts with K + by a single-phase insertion reaction: CuHCF electrodes are promising for grid-scale energy storage applications because of their ultra-long cycle life (83% capacity retention after 40,000 cycles), high power (67% capacity at 80C), high energy efficiency and, potentially, a very low cost. An anode to operate in the same electrolyte as the CuHCF cathode must be chemically stable in acidic solutions (pH 1–2) [16] and preferably have a potential near −0.1 V versus the standard hydrogen electrode (SHE), the thermodynamic limit for water decomposition at this pH. In addition, a useful anode must have a very long cycle life and high-rate capability to match the remarkable properties of the CuHCF cathode. In addition to K + , CuHCF can also react with alkali ions, such as Li + and Na + , so an anode capable of reacting with any of these ions could be used [17] . An intuitive choice would be another Prussian Blue analogue with a reaction potential near the SHE. However, the reduction of Prussian Blue to Everitt's Salt occurs at too high a potential (0.45 V versus SHE) [18] and other Prussian Blue analogues containing electrochemically active hexacyanomanganate and hexacyanochromate are chemically unstable [19] . In this work, we describe a new class of anodes that are compatible with our open-framework CuHCF materials in aqueous electrolytes. These anodes are based on a hybrid electrode that operates by a new fundamental concept; that is, by combining an electrode material (polypyrrole, PPy), which is capable of a faradaic reaction at a fixed potential with a capacitive electrode (activated carbon, AC), the potential of the entire electrode can be controlled. Fundamentally different from traditional capacitive and battery electrodes, our new hybrid electrode has the high-rate capability of an ultra-capacitor, but with the well-defined potential of a battery electrode. This hybrid electrode has an attractive open-circuit potential (OCP), tunable to −0.2 V versus SHE, a shallow charge/discharge profile and low self-discharge. Furthermore, we demonstrate that a full cell with this hybrid anode and a CuHCF cathode gives performance which is promising for grid-scale stationary storage applications, such as high power and energy efficiency, and a lifetime of thousands of cycles. Hybrid-AC/PPy anode Electrochemical double-layer capacitors (EDLCs) are known to operate in a variety of aqueous and organic electrolytes, and can have extremely high specific power and cycle life [20] . However, the cycling of an EDLC electrode proceeds by the physical formation and dispersal of a double layer of charge at the electrode surface with no faradaic reaction involving the bulk material [21] . This results in very low specific capacity and deleterious self-discharge [2] . Another drawback is that the potential of a capacitive electrode varies nearly linearly with charge state, so capacitors offer useful energy and power only at shallow discharge [21] . In addition, in the case of AC, negatively charged surface groups that improve hydrophilicity also raise the OCP in aqueous electrolytes to above 0.3 V versus SHE, which is too high for a useful anode with a CuHCF cathode [22] , [23] . One benefit of using AC as an anode in aqueous electrolytes is its suppression of H 2 evolution at low potentials [24] , but its low capacity, steep discharge profile and high OCP limit its practicality. The electrochemical properties of conductive polymers such as PPy have been explored in both organic and aqueous electrolytes [25] , [26] . PPy is very insoluble in aqueous electrolytes [26] . Its electrochemical cycling proceeds by a p-type doping/de-doping process: Anions from the electrolyte coordinate to the PPy chains during oxidation, and they are released during reduction [27] . The reduction and oxidation of the polymer could also be balanced by smaller ions, such as H 3 O + in acidic aqueous electrolytes, which can fit into the existing paracrystalline lattice as previously demonstrated in the case of poly(3,4-ethylenedioxythiophene) [28] . The reaction potential of PPy depends on the particular doping anion [29] , but is typically near 0 V versus SHE, making it attractive for use as an anode in aqueous cells (Fig. 2a). A PPy anode was recently paired with LiCoO 2 in an aqueous lithium-ion battery, but its low electronic conductivity upon reduction severely limited the rate capability, energy efficiency and cycle life of the cell [27] . Although it has a high theoretical specific capacity of 82 mAh g −1 (ref. 30 ), PPy alone cannot be used as a high-performance anode. Here we combine an EDLC with PPy into a hybrid electrode synergistically. We explore using PPy as a minor additive component to define the potential of AC, whereas most of the charge storage is by AC. For this purpose, PPy nanoparticles ( Fig. 1d,f ) were synthesized by oxidative polymerization of pyrrole [31] . This hybrid anode combines the fast kinetics of AC and the low reaction potential of fully reduced PPy. In practice, this combination of properties can be achieved simply by intimately mixing AC with small amounts of reduced PPy in a single-electrode structure. This occurs because the OCP of AC and other EDLCs depends on its surface charge density and, therefore, is well-defined. Thus, in the case of electrical contact between AC and a material having a distinct redox couple, the OCP of the AC will be fixed to the potential of that redox couple. So, in the case of an AC/PPy electrode, the OCP is determined by the potential of the PPy component despite its small quantity. The as-synthesized PPy powder is fully oxidized (doped) and has a high OCP of 0.5 V versus SHE. An electrode containing doped PPy and AC will also have a high OCP as explained above. Using a previously reported method for the reduction of pure PPy powder by sodium borohydride (NaBH 4 ), electrodes containing both AC and PPy can be reduced, resulting in an OCP of −0.1 V versus SHE ( Fig. 2 ) [32] . 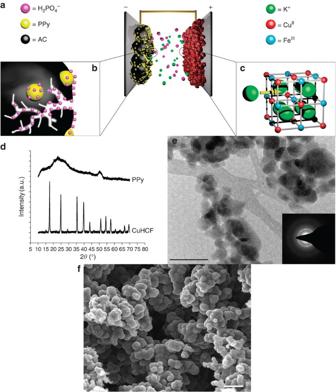Figure 1: Full cell schematic and physical characterization of the electrode materials. (a) Schematic diagram of full cell device. In the PPy/AC negative electrode (b), the reduced PPy particles fix the open-circuit potential close to the lower-stability limit of the electrolyte, whereas the charge is stored in the electrical double layer at the high-surface AC. The CuHCF-positive electrode (c) has the open-framework Prussian Blue crystal structure, in which transition metal ions are linked by a face-centered cubic framework of cyanide groups. In the case of CuHCF, octahedral hexacyanoferrate groups form a framework with sixfold nitrogen-coordinated copper. The framework contains large interstices, known as the 'A Sites', which may contain zeolitic water or mobile, hydrated alkali ions. Hydrated ions may readily pass between one A Site and the next through channels in the <100> directions. This three-dimensional network of A Sites and channels allows for rapid transport of K+through the material without disturbing the framework. Zeolitic water is omitted for clarity. (d) X-ray diffraction patterns of CuHCF and PPy. Bulk synthesis of CuHCF at room temperature by co-precipitation results in highly crystalline material. PPy particles are about 200–400 nm. At 2θ=11.5° and 26°, there are two broad peaks in the XRD pattern, indicating the existence of a short-range order and an ordered structure between the PPy chains. (e) Transmission electron microscope photo of CuHCF shows polydispersed 20–50 nm particles. Scale bar equals 100 nm. (f) Scanning electron microscope photo of PPy shows particles of the order of 200–400 nm. Scale bar equals 2 μm. Figure 1: Full cell schematic and physical characterization of the electrode materials. ( a ) Schematic diagram of full cell device. In the PPy/AC negative electrode ( b ), the reduced PPy particles fix the open-circuit potential close to the lower-stability limit of the electrolyte, whereas the charge is stored in the electrical double layer at the high-surface AC. The CuHCF-positive electrode ( c ) has the open-framework Prussian Blue crystal structure, in which transition metal ions are linked by a face-centered cubic framework of cyanide groups. In the case of CuHCF, octahedral hexacyanoferrate groups form a framework with sixfold nitrogen-coordinated copper. The framework contains large interstices, known as the 'A Sites', which may contain zeolitic water or mobile, hydrated alkali ions. Hydrated ions may readily pass between one A Site and the next through channels in the <100> directions. This three-dimensional network of A Sites and channels allows for rapid transport of K + through the material without disturbing the framework. Zeolitic water is omitted for clarity. ( d ) X-ray diffraction patterns of CuHCF and PPy. Bulk synthesis of CuHCF at room temperature by co-precipitation results in highly crystalline material. PPy particles are about 200–400 nm. At 2 θ =11.5° and 26°, there are two broad peaks in the XRD pattern, indicating the existence of a short-range order and an ordered structure between the PPy chains. ( e ) Transmission electron microscope photo of CuHCF shows polydispersed 20–50 nm particles. Scale bar equals 100 nm. ( f ) Scanning electron microscope photo of PPy shows particles of the order of 200–400 nm. Scale bar equals 2 μm. 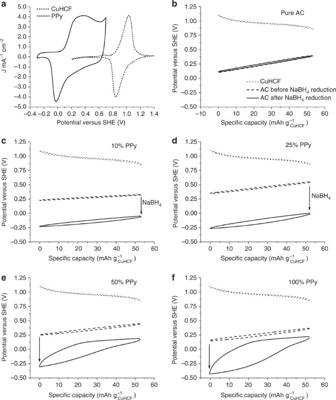Figure 2: Hybrid AC/PPy anode. (a) Cyclic voltammetry scans of CuHCF and PPy at 1 mV s−1scan rate, (b–f) galvanostatic cycling of PPy/AC anodes at different ratios of PPy/AC at 1C rate. PPy/AC anodes before (---) and after (—) the NaBH4chemical reduction step with 0.1 M NaBH4and CuHCF cathode (···). The specific capacity values have been normalized by the mass of cathode, which is on the order of 10 mg cm−2, whereas the anode mass is on the order of 50 mg cm−2. The open-circuit potentials of the electrodes are on the right-end side for the cell cycling started from full discharge. Full size image Figure 2: Hybrid AC/PPy anode. ( a ) Cyclic voltammetry scans of CuHCF and PPy at 1 mV s −1 scan rate, ( b – f ) galvanostatic cycling of PPy/AC anodes at different ratios of PPy/AC at 1C rate. PPy/AC anodes before (---) and after (—) the NaBH 4 chemical reduction step with 0.1 M NaBH 4 and CuHCF cathode (···). The specific capacity values have been normalized by the mass of cathode, which is on the order of 10 mg cm −2 , whereas the anode mass is on the order of 50 mg cm −2 . The open-circuit potentials of the electrodes are on the right-end side for the cell cycling started from full discharge. Full size image Effect of the PPy/activated-carbon ratio To look for the ideal PPy percentage that can define the OCP of −0.1 V versus SHE while storing charge in the AC component, we have carried out experiments with five different PPy percentages: 0, 10, 25, 50 and 100%. We have found that hybrid AC/PPy electrodes have very interesting electrochemical properties, depending on the percentage of PPy. First, all the electrodes with or without PPy have high OCP of about 0.4 V versus SHE before the NaBH 4 reduction treatment. These electrodes do not have an attractive voltage to pair with CuHCF. Second, after NaBH 4 reduction treatment, all the electrodes containing PPy ( Fig. 2c–f ) have a significantly lower OCP of −0.25 V versus SHE. This OCP is low enough for practical use with the CuHCF cathode. In comparison, pure AC electrodes do not undergo faradaic reactions, and their OCP is not lowered by NaBH 4 chemical reduction ( Fig. 2b ). This difference is clearly due to the reduction of PPy by NaBH 4 , but the NaBH 4 does not change the AC. Third, as the fractional PPy content of the hybrid electrode increases from 10 to 100%, the voltage hysteresis observed during cycling at a 1C rate grows dramatically ( Fig. 2c–f ). This occurs because fully reduced PPy is electronically insulating [33] . Hybrid electrodes with a PPy content as low as 10% result in the same low, stable OCP of a pure PPy electrode. AC/PPy electrodes of even lower PPy content did not have stable OCPs (data not shown). The optimal PPy content was found to be 10%, as this quantity was sufficient to maintain a stable, low OCP and cycling potential without limiting the high efficiency of the AC. CuHCF chemical reduction The novel AC/PPy hybrid anode can be combined with a wide variety of cathodes to produce full cell batteries. The hybrid anode with 10% PPy is used for the following full cell study. Here, we demonstrate its use in cells that contain CuHCF cathodes. When constructing a full cell with a CuHCF cathode and an AC/PPy hybrid anode, additional complications must be addressed. First, the two electrodes in a full cell must have appropriate initial charge states. The AC/PPy anode was chemically reduced so that its OCP was equal to the reaction potential of fully reduced PPy. Previous syntheses of CuHCF resulted in a material with a fractional initial charge state, because fully oxidized CuHCF has a potential so high that it can be reduced by water. To address this concern, a reductive titration method was developed to controllably reduce CuHCF to a desired oxidation state and OCP using sodium thiosulfate (Na 2 S 2 O 3 ; Fig. 3a ). 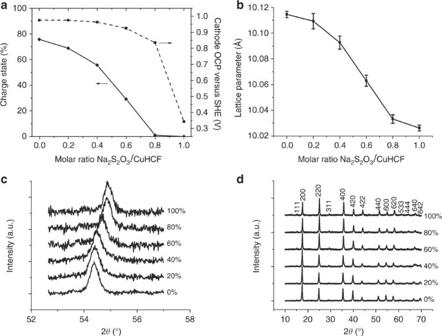Figure 3: CuHCF chemical reduction. (a) Charge state of the CuHCF and cathode open-circuit potential as a function of the molar ratio Na2S2O3added/CuHCF. The decrease in the lattice parameter of CuHCF with chemical reduction (b) is illustrated by the shift of the <600> diffraction peak to smaller angles (c,d). The lattice parameters indare the average calculated for ten diffraction peaks. The error bars are ±1 s.d. around this value. In the case of full reduction of CuHCF, this reaction may be described by: Figure 3: CuHCF chemical reduction. ( a ) Charge state of the CuHCF and cathode open-circuit potential as a function of the molar ratio Na 2 S 2 O 3 added/CuHCF. The decrease in the lattice parameter of CuHCF with chemical reduction ( b ) is illustrated by the shift of the <600> diffraction peak to smaller angles ( c , d ). The lattice parameters in d are the average calculated for ten diffraction peaks. The error bars are ±1 s.d. around this value. Full size image Before the addition of any Na 2 S 2 O 3 , CuHCF is about 80% charged, so the addition of Na 2 S 2 O 3 in a ratio of Na 2 S 2 O 3 :CuHCF of 0.8 results in full reduction. CuHCF can intercalate either K + or Na + . Though both K + and Na + are present during the reductive titration, CuHCF intercalates only K + because of its higher-equilibrium reaction potential [14] , and the OCPs observed after chemical reduction correspond to the potential of CuHCF observed at the same charge state during electrochemical cycling. Electrochemical reduction of CuHCF and other Prussian Blue analogues results in a decrease in lattice parameter, as the iron–carbon bond in Fe(CN) 6 shortens by 0.05 Å ( Fig. 3b–d ) [34] . Full cell assembly Full cells were assembled with electrodes in their discharged states. Fully reduced CuHCF that was treated with Na 2 S 2 O 3 in a 0.8:1 molar ratio was used as the cathode. The anode was 10% PPy/AC, pretreated with NaBH 4 . It is initially counterintuitive to consider a reduced anode to be in a discharged state; but as previously noted, the only role of the PPy additive is to fix the OCP of the electrode at the desired value; to have low hysteresis and therefore high energy efficiency, the contribution of the doping/dedoping process of PPy to the electrode capacity must be negligible. For this reason, the anode was cycled over a potential range below that of the dedoping process of the PPy additive. In the first cycle, the battery is charged from its initial state, meaning that potassium ions are removed from the CuHCF framework at the cathode and that a charge double layer is formed at the anode. Another challenge for the development of a full cell using CuHCF and AC/PPy electrodes is the disparity in the specific capacities of the electrodes. The double-layer capacitance in aqueous electrolytes is 10–50 μF cm −2 , so EDLCs must be cycled over wide potential ranges to achieve appreciable capacity [21] . Aqueous batteries have low voltages that are limited by water decomposition. A flat full-cell voltage profile is desirable because the stored energy scales with voltage, and the output power scales with the square of the voltage. If the voltage varies greatly with charge state, some of the charge is available only at voltages too low to provide practical values of energy and power. Therefore, electrodes in aqueous batteries should preferably be cycled over limited potential ranges so that the full discharge of the device produces usable energy. In the case of capacitive electrodes, the same charge can be accessed in a smaller potential window if a larger exposed surface and, therefore, a larger mass is used. The CuHCF versus AC/PPy cells described here contained a 10 mg cm −2 , 1 cm 2 CuHCF cathode and a 50 mg cm −2 , 2 cm 2 AC/PPy anode, resulting in a cathode/anode mass loading ratio of 1:10. In full cells, the electrolyte must also be optimized to allow reversible cycling of both electrodes. Previous studies of CuHCF and other Prussian Blue analogues used electrolytes with pH between 2 and 4 [16] . In the full cells reported here, CuHCF was found to be most chemically stable at pH 1. Full cell cycling with potential cut-off values of 0.85 and 1.1 V for the CuHCF cathode resulted in a full cell voltage range of 1.4–0.9 V ( Fig. 4a,c ) and a maximum specific capacity of 54 mAh g −1 CuHCF. Because of its high mass loading, the potential of the AC/PPy anode changes by only 250 mV during cycling, so the changes in the potentials of the two electrodes contribute similarly to the slope of the full cell voltage profile. The potential hysteresis of the anode is higher than that of the cathode because of its high mass loading (50 mg cm −2 ) and thickness (1 mm). At a 10C rate, 82% of the maximum specific capacity is retained, with a round-trip energy efficiency of 92% ( Fig. 4b ), and at a rate of 50C 33% of the maximum specific capacity is observed at an efficiency of 79%. Cycling was highly reversible, with zero-capacity loss after 1,000 cycles at a 10 C rate, and the coulombic efficiency was 99.9% ( Fig. 4d ). 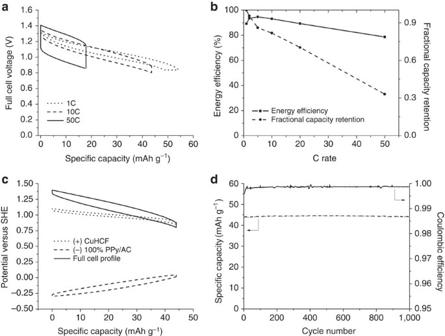Figure 4: Full cell electrochemical characterization. (a) Full cell potential profiles at different C rates (1C, 10C, 50C). (b) Energy efficiency and fractional capacity retention as a function of the C rate. (c) Potential profiles of CuHCF-positive electrode, 10% PPy/AC anode-negative electrode and full cell profile at 10C. (d) Cycling of the CuHCF–10% PPy/AC cell at a rate of 10C showed no capacity loss after 1,000 cycles and a coulombic efficiency of 99.9%. Figure 4: Full cell electrochemical characterization. ( a ) Full cell potential profiles at different C rates (1C, 10C, 50C). ( b ) Energy efficiency and fractional capacity retention as a function of the C rate. ( c ) Potential profiles of CuHCF-positive electrode, 10% PPy/AC anode-negative electrode and full cell profile at 10C. ( d ) Cycling of the CuHCF–10% PPy/AC cell at a rate of 10C showed no capacity loss after 1,000 cycles and a coulombic efficiency of 99.9%. Full size image The high capacity retention and rate capability of the CuHCF versus AC/PPy full cells result in high specific power. The average specific power during discharge at a 10C rate during cycling between 1.4 and 0.9 V was 45 W kg −1 on the basis of the electrode active materials, and a maximum specific power of nearly 100 W kg −1 was achieved at 20C. The specific energy of the cells reported here was about 5 W h kg −1 , lower than the conventional lithium-ion, lead acid and NiMH batteries. However, as the discharge voltage was limited to 0.9 V, all of the specific energy of the cell can be practically used. The specific power and energy of the CuHCF versus AC/PPy cell is limited by the high mass loading of the anode. In this study, inexpensive, commercially available AC that was hydrophobic and, therefore, had a low effective surface area in water was used. Reducing the anode mass loading by 50% simply by using a more hydrophilic AC with a higher-effective specific surface area would nearly double the specific energy and power. Also, the cells reported here used a flooded geometry that resulted in excessive electrolyte resistance. The use of pressed cells will significantly improve energy efficiency and specific power at high cycling rates. In summary, novel aqueous potassium ion batteries using an open-framework crystal structure CuHCF cathode and a new type of fixed-potential capacitive anode were demonstrated to have long cycle life, high power and high efficiency. The CuHCF cathode is synthesized by a simple, scalable, room-temperature chemical co-precipitation method. The anode combines commercially available, inexpensive AC with PPy, which may be synthesized in bulk near room temperature. The electrodes operate in safe, inexpensive aqueous electrolytes. The performance, scalability and safety of these cells make them desirable for stationary storage applications, including the smoothing of intermittent solar and wind power. The addition of electrochemically active additives with fixed potentials to capacitive electrodes may be employed in a wide variety of devices in which one or both of the electrodes is of this kind. Study of other types of devices using one or two EDLC/additive hybrid electrodes is underway. CuHCF synthesis Preparation of nanoparticulate CuHCF was based on our recently reported synthesis [12] . Briefly, equal volumes of 40 mM Cu(NO 3 ) 2 (Alfa Aesar) and 20 mM K 3 Fe(CN) 6 (Sigma Aldrich) were combined by simultaneous, dropwise addition into water under vigorous stirring. An excess of Cu +2 is necessary for precipitation and particle growth. All of the Fe(CN) 6 is oxidized initially, but fully charged CuHCF has a potential high enough to oxidize water. Thus, spontaneous partial reduction of CuHCF occurs, resulting in a fractional initial charge state, typically between 50 and 80% of total capacity. Five minutes after complete addition of the CuHCF precursors, 0.1 M Na 2 S 2 O 3 was added until a desired molar ratio of Fe III (CN) 6 −3 to S 2 O 3 −2 was reached. The colour of CuHCF changed from a dingy yellow to deep claret upon addition of Na 2 S 2 O 3 , indicating a successful reduction. The CuHCF was filtered, washed with water and dried in vacuum at room temperature. Slurries containing CuHCF, amorphous carbon (Super P Li), poly(vinylidene) difluoride (Kynar HSV900) and graphite (Timcal KS6) in a ratio of 80:9:9:2 were prepared by grinding these materials by hand and then dispersing them in 1-methyl-2-pyrrolidinone. Electrodes with mass loadings of about 10 mg cm −2 CuHCF were prepared by spreading the slurry on a carbon cloth current collector (Fuel Cell Earth). The electrodes were dried in vacuum at 60 °C for 1 h. PPy synthesis PPy was prepared by chemical oxidative polymerization of the corresponding monomer (pyrrole) in an aqueous medium as described elsewhere [31] . Pyrrole (0.03 mol, 2 ml) was dispersed in 150 ml of de-aerated (N 2 ) cold water (0 °C). Anhydrous Na 2 S 2 O 8 (oxidant; 6.61 g, 0.03 mol) was dissolved in 50 ml of cold (0 °C) water in a reaction vessel containing a magnetic stirring bar and added dropwise into the stirred pyrrole solution. The reaction was carried out for 8 h at 0 °C with moderate stirring. The precipitated PPy was filtered off, washed with distilled water and dried in vacuum at 60 °C for 8 h. The black PPy slurries containing 10% poly(vinylidene) difluoride and 90% active material, with AC and PPy in the desired ratio, were prepared in 1-methyl-2-pyrrolidinone. Negative electrodes with mass loadings of 50 mg cm −2 were prepared by the method used for the CuHCF-positive electrodes. PPy chemical reduction The chemical reduction of the PPy was carried out by immersing the electrodes for 20 min in a 0.1 M solution of NaBH 4 as previously described in the paper by Bengoechea et al . [32] The reduction process may also be performed on the raw PPy powder, but this could lead to material degradation if stored in air. Electrochemical cell set-up Flooded full cells containing a CuHCF cathode, an AC/PPy anode, a 1 M potassium phosphate buffer at pH 1 and a Ag/AgCl reference electrode were prepared in a nitrogen-filled glovebox. The AC/PPy electrode is sensitive to oxidation, so the cell must be kept oxygen free to achieve efficient anode cycling at potentials below the SHE. How to cite this article: Pasta, M. et al . A high-rate and long cycle life aqueous electrolyte battery for grid-scale energy storage. Nat. Commun. 3:1149 doi: 10.1038/ncomms2139 (2012).